Intercalation and delamination of layered carbides and carbonitrides Intercalation and delamination of two-dimensional solids in many cases is a requisite step for exploiting their unique properties. Herein we report on the intercalation of two-dimensional Ti 3 C 2 , Ti 3 CN and TiNbC—so called MXenes. Intercalation of hydrazine, and its co-intercalation with N , N -dimethylformamide, resulted in increases of the c -lattice parameters of surface functionalized f-Ti 3 C 2 , from 19.5 to 25.48 and 26.8 Å, respectively. Urea is also intercalated into f-Ti 3 C 2 . Molecular dynamics simulations suggest that a hydrazine monolayer intercalates between f-Ti 3 C 2 layers. Hydrazine is also intercalated into f-Ti 3 CN and f-TiNbC. When dimethyl sulphoxide is intercalated into f-Ti 3 C 2 , followed by sonication in water, the f-Ti 3 C 2 is delaminated forming a stable colloidal solution that is in turn filtered to produce MXene ‘paper’. The latter shows excellent Li-ion capacity at extremely high charging rates. A unique characteristic of layered materials is their ability to accommodate various ions and molecules between their layers, a phenomenon known as intercalation. Intercalation compounds of inorganic hosts (graphite, clays, di-chalcogenides and others) have also gained renewed interest owing to their unique chemical and physical properties [1] , [2] , [3] , [4] , [5] , [6] . De-intercalation of those compounds under certain conditions (such as thermal shock) as well as sonication or volume expansion reactions in the interlayer space lead to the formation of widely used exfoliated graphite [7] , [8] , [9] , [10] , [11] and two-dimensional (2D) materials with unusual electronic properties [12] , [13] , [14] , [15] . Recently, a large family of 2D materials, labelled MXenes—produced by the extraction of the A-element from the layered ternary carbides, such as Ti 3 AlC 2 and other MAX phases [16] , where M is an early transition metal, A is an A group element, and X is C or N—was discovered [17] , [18] . The MXenes produced to date, viz., Ti 3 C 2 (ref. 17 ), Ti 2 C, Ta 4 C 3 , (Ti 0.5 Nb 0.5 ) 2 C, (V 0.5 Cr 0.5 ) 3 C 2 and Ti 3 CN (ref. 18 ) are, in many aspects, graphene-like, forming stacks of sheets and scrolls. They also are good electrical conductors [17] , [18] , [19] , [20] , [21] and are predicted to have high elastic moduli. [22] Electrochemical intercalation of Li ions between the MXene sheets renders these solids promising materials for Li-ion battery anodes and hybrid electrochemical capacitors [23] , [24] , [25] . However, up to now there have been no reports of the chemical intercalation or large-scale delamination of MXenes or any other transition metal carbides. It is important to note at the outset that the 2D MXene surfaces are not M-terminated, but covered with oxygen-containing groups, such as OH, and fluorine (F) introduced after etching with aqueous hydrofluoric acid (HF) [17] . The chemistry of exfoliated MXene produced by HF etching of Ti 3 AlC 2 is much closer to Ti 3 C 2 (OH) x O y F z than to the idealized structure of a pure carbide layer Ti 3 C 2 . Henceforth, and for brevity’s sake, f-Ti 3 C 2 will be used instead of the more cumbersome Ti 3 C 2 (OH) x O y F z . The original aim of this work was to reduce the f-Ti 3 C 2 surfaces to create Ti-terminated surfaces that theory predicts would be magnetic [25] . A perusal of the graphene literature made it clear that hydrazine monohydrate N 2 H 4 ·H 2 O (HM) dissolved in N , N -dimethylformamide (DMF) is the reactant of choice [26] . Since in our case, HM was found to primarily act as an intercalant rather than a reducing agent, the research objectives were redirected towards intercalation and delamination of MXenes. Furthermore, as the layered structures of the MXenes retain some similarities to clays [17] , we reviewed the intercalation chemistries of the latter. Numerous compounds, such as formamide and its derivatives, dimethyl sulphoxide (DMSO), urea and long-chain alkylamines, among others have been shown to intercalate clays [27] . For clays, HM is probably the most common intercalant; its intercalation results in the increase of kaolinite’s c -lattice parameter ( c- LP) from 7.2 to 10.3–10.4 Å (refs 27 , 28 , 29 ). Here we report, for the first time, on the intercalation of f-Ti 3 C 2 with urea, HM, HM dissolved in DMF and DMSO. Importantly, intercalation of DMSO enabled us to delaminate stacked f-Ti 3 C 2 layers into separate 2D MXene sheets. We also show that HM intercalates Ti 3 CN and TiNbC. Intercalation of MXenes A schematic of MXene intercalation is shown in Fig. 1a . X-ray diffraction (XRD) showed that after intercalation with HM and/or DMF, the (000l) peaks were still present, but shifted to lower 2θ angles ( Fig. 1b and Supplementary Fig. S1 ). 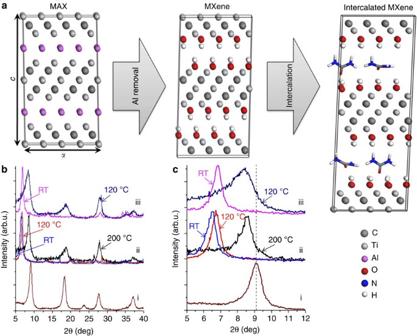Figure 1: Evidence of MXene intercalation. (a) Schematic of synthesis and intercalation of f-Ti3C2. First, the Al layer is removed from the corresponding MAX phase in 50% aqueous HF. The f-MXene is then treated with an intercalant (urea is shown as an example) yielding intercalation compounds. (b) XRD patterns of f-Ti3C2: (i) as received, before any treatment, (ii) after HM in DMF treatment, washed with DMF, (iii) after HM treatment, washed with ethanol and dried in different conditions. (c) Zoom-ins ofbin the 5–12° 2θ range showing (0002) peaks. Table 1 summarizes the c -LPs values for f-Ti 3 C 2 treated with HM and HM in DMF. The initial c -LP was 19.5±0.1 Å, a value that does not change much with post-intercalation drying ( Table 1 ). After exposure to HM or HM in DMF at 80 °C for 24 h, the c -LPs increased to 25.48±0.02 and 26.8±0.1 Å, respectively. The larger c -LP increase in the latter case points to a synergistic effect when HM is dissolved in DMF before intercalation. Figure 1: Evidence of MXene intercalation. ( a ) Schematic of synthesis and intercalation of f-Ti 3 C 2 . First, the Al layer is removed from the corresponding MAX phase in 50% aqueous HF. The f-MXene is then treated with an intercalant (urea is shown as an example) yielding intercalation compounds. ( b ) XRD patterns of f-Ti 3 C 2 : (i) as received, before any treatment, (ii) after HM in DMF treatment, washed with DMF, (iii) after HM treatment, washed with ethanol and dried in different conditions. ( c ) Zoom-ins of b in the 5–12° 2θ range showing (0002) peaks. Full size image Table 1 Summary of the c -LPs, in Å, values for non-intercalated f-Ti 3 C 2 and f-Ti 3 C 2 treated with HM and HM in DMF. Full size table When the HM-intercalated powders were heated to 120 °C in a vacuum oven, the c -LP decreased from 25.48±0.02 to 20.6±0.3 Å, signifying that the intercalation process is essentially reversible. Heating powders intercalated with HM and DMF under the same conditions resulted in small increases in the 2θ angles ( Fig. 1b-ii ). Thus, the HM/DMF combination is more resistant to de-intercalation than HM alone, possibly because of the higher boiling point of DMF (153 °C) compared with that of HM (114 °C). However, when f-Ti 3 C 2 intercalated with HM and DMF was vacuum dried at 200 °C, the c -LP decreased to 20.1±0.5 Å. X-ray photoelectron spectroscopy (XPS) ( Supplementary Fig. S2 ) provides further evidence of intercalation. As previously reported [17] , exfoliated f-Ti 3 C 2 showed the presence of Ti–C and Ti–O bonds, as well as OH groups, suggested by the presence of a O1s peak around 532 eV (see Supplementary Materials for more details). A N1s signal was also observed around 400 eV in XPS spectra of f-Ti 3 C 2 treated with HM and HM/DMF (insets in Supplementary Figs S2a,b , respectively). No nitrogen peaks were detected in f-Ti 3 C 2 before intercalation. Scanning electron microscopy (SEM) images of f-Ti 3 C 2 , before and after HM treatment in DMF at 80 °C for 24 h, shown in Fig. 2a , respectively, confirm that: (i) the MXene remains exfoliated after intercalation, and, (ii) the multilayers thicken ( Fig. 2b ) apparently by gluing individual monolayers together, forming 20–50-nm-thick lamellas. Note that the absence of XRD peaks corresponding to a c -LP of 19.5 Å ( Fig. 1b-i ) implies that intercalation was essentially complete. 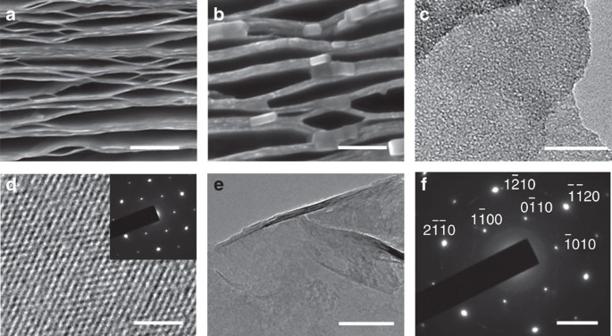Figure 2: Morphology characterization. (a,b) SEM images before (a) and after (b) intercalation of f-Ti3C2with HM and DMF (24 h at 80 °C), respectively. (c,d) TEM (c) and high-resolution electron microscopy (d) images (inset shows selected area electron diffraction (SAED) pattern) before intercalation. (e,f) TEM image (e) and SAED pattern (f) of intercalated f-Ti3C2. Scale bars, 200 nm ina,b; 10 nm inc; 2 nm ind; 40 nm ine; and 4 nm−1inf. Figure 2: Morphology characterization. ( a , b ) SEM images before ( a ) and after ( b ) intercalation of f-Ti 3 C 2 with HM and DMF (24 h at 80 °C), respectively. ( c , d ) TEM ( c ) and high-resolution electron microscopy ( d ) images (inset shows selected area electron diffraction (SAED) pattern) before intercalation. ( e , f ) TEM image ( e ) and SAED pattern ( f ) of intercalated f-Ti 3 C 2 . Scale bars, 200 nm in a , b ; 10 nm in c ; 2 nm in d ; 40 nm in e ; and 4 nm −1 in f . Full size image Transmission electron microscopy (TEM) images and corresponding selected area electron diffraction patterns of f-Ti 3 C 2 intercalated with HM in DMF at 80 °C for 24 h ( Fig. 2e ) showed that the basal planes’ hexagonal structure remains unchanged (compare inset in Fig. 2d with Fig. 2f ) after intercalation [17] . The interplanar spacing in intercalated f-Ti 3 C 2 —2.648 Å for ( ) and 1.540 Å for ( )—results in an a- LP of 3.057 Å, in excellent agreement with the a- LP of f-Ti 3 C 2 before intercalation and that of the Ti 3 AlC 2 , viz., 3.058 Å [17] . To demonstrate that intercalation is a general phenomenon rather than the exclusive property of f-Ti 3 C 2 , the MXenes Ti 3 CN and TiNbC were also treated with HM. Similar to f-Ti 3 C 2 , the shift of the major XRD peak of these MXenes to lower 2θ values ( Supplementary Fig. S3 ) confirmed their intercalation. It is thus reasonable to conclude that f-MXenes—like other layered materials—can be readily intercalated by many different compounds. In addition, the electrical resistivities of non-intercalated MXenes and MXenes treated with HM were measured. The resistivity values of all intercalated samples were higher than those of non-intercalated MXenes presumably owing to the increase of their c -LPs after intercalation ( Supplementary Table S1 ). The differences in the magnitudes of the resistivity increases for different intercalated MXenes, at relatively the same expansion, can be partially explained by the different number of MXene atomic layers. In case of M 3 X 2 (five atomic layers), the resistivity increases by an order of magnitude, whereas an increase by two orders is observed for the M 2 C (three atomic layers) compounds. Molecular dynamics (MD) simulations To further our understanding of the structure of intercalated MXene, MD simulations of N 2 H 4 inserted between OH-terminated Ti 3 C 2 layers were carried out ( Fig. 3a ). MXene supercells (4 × 2 × 1 (a × b × c)) with N 2 H 4 uniformly spaced between the MXene layers at different concentrations were constructed for MD studies. A detailed description of the simulations is provided in the Supplementary Methods . With no N 2 H 4 molecules, the MD-computed c -LP value is reasonably close to the experimental result ( Table 1 ) and density functional theory (DFT)-calculated values [17] . When two N 2 H 4 molecules are introduced (one into each interlayer space), the c -LP sharply jumps to 24.93±0.01 Å ( Fig. 3a ). Further increase of the number of N 2 H 4 molecules results in only slightly changed c- LPs (from 24.93 to 25.31 Å), corresponding to N 2 H 4 monolayer formation ( Fig. 3a ) within the widened interlayer MXene space. With six N 2 H 4 molecules per supercell (three inside each interlayer space as shown in Fig. 3b ), the intercalant monolayer formation is complete and the introduction of the next pair of N 2 H 4 molecules results in a second sharp increase of c -LP from 25.31±0.04 Å (six N 2 H 4 molecules) to 27.28±0.03 Å (eight N 2 H 4 molecules) as shown in Fig. 3a , which is an evidence for the onset for the formation of a second intercalant layer (see also MD snapshot in Supplementary Fig. S4a ). 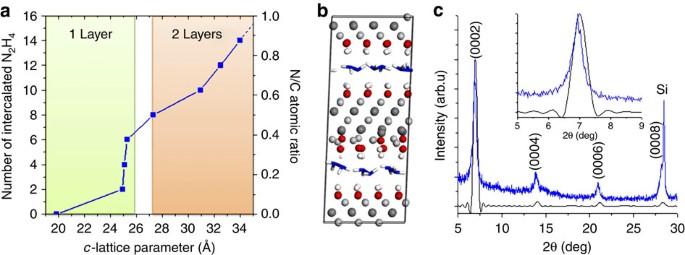Figure 3: Molecular dynamic simulations of OH-terminated Ti3C2intercalated with hydrazine. (a) Change in f-MXenec-LP as a function of the number of N2H4intercalated molecules. As the latter is increased, first a monolayer of N2H4molecules is formed, corresponding to the N/C ratio~0.4 (c=25–26 Å). Further increase in the number of N2H4-intercalated molecules results in the onset of the second layer formation, which is not complete up to the maximum N/C ratio employed in the simulations (N/C=0.875). (b) Molecular dynamic snapshot of hydrazine intercalated MXene for N/C ratio 0.375 (six N2H4per a 4 × 2 × 1 MXene supercell) showing a nearly complete N2H4monolayer. For colour coding of the elements, please seeFig. 1a. (c) Comparison of simulated (black) and experimental (blue) XRD patterns of N2H4intercalated OH-terminated Ti3C2. Figure 3: Molecular dynamic simulations of OH-terminated Ti 3 C 2 intercalated with hydrazine. ( a ) Change in f-MXene c -LP as a function of the number of N 2 H 4 intercalated molecules. As the latter is increased, first a monolayer of N 2 H 4 molecules is formed, corresponding to the N/C ratio~0.4 ( c =25–26 Å). Further increase in the number of N 2 H 4 -intercalated molecules results in the onset of the second layer formation, which is not complete up to the maximum N/C ratio employed in the simulations (N/C=0.875). ( b ) Molecular dynamic snapshot of hydrazine intercalated MXene for N/C ratio 0.375 (six N 2 H 4 per a 4 × 2 × 1 MXene supercell) showing a nearly complete N 2 H 4 monolayer. For colour coding of the elements, please see Fig. 1a . ( c ) Comparison of simulated (black) and experimental (blue) XRD patterns of N 2 H 4 intercalated OH-terminated Ti 3 C 2 . Full size image The experimental c -LP value for N 2 H 4 -intercalated f-MXene ( c =25.48 Å, Table 1 ) corresponds to an MD-derived N/C ratio ~0.39 ( Fig. 3a ), that is, to the formation of a nearly complete monolayer of N 2 H 4 molecules in each MXene interlayer space. The N/C ratio, determined by XPS for the HM-intercalated MXene dried at room temperature, is 0.37, in very good agreement with the value deduced from the MD simulations (~0.4) for the situation with a nearly complete monolayer of N 2 H 4 molecules ( Figs 3a ). Furthermore, the computed XRD pattern for the system of this composition is close to the one measured experimentally ( Fig. 3c ). Delamination of MXene We also tried to intercalate thiophene, ethanol, acetone, tetrahydrofuran, formaldehyde, chloroform, toluene, hexane, DMF, DMSO and urea into f-Ti 3 C 2 at room temperature. Of these, only DMSO and urea resulted in an increase in the c -LPs from 19.5±0.1 Å to 35.04±0.02 Å and 25.00±0.02 Å, respectively ( Supplementary Fig. S5 ). It follows that DMF only intercalates into f-Ti 3 C 2 in the presence of HM. Coincidentally or not, of the aforementioned list of organic compounds, only DMSO and urea intercalate kaolinite [27] , [30] . XRD patterns, taken 3 weeks after the initial DMSO intercalation ( Supplementary Fig. S5-ii , red curve), showed an even larger downshift of the (0002) peak positions corresponding to a c -LP of 44.8±0.1 Å. Based upon this result, combined with the observation that DMSO-intercalated f-MXene powders are highly hygroscopic and become increasingly wet when stored in air over a few weeks, it is reasonable to assume that, over time, co-intercalation or capillary condensation of water from ambient air into the interlayer space occurred. This discovery, in turn, was exploited to fully exfoliate—what we term delaminate herein (see Supplementary Fig. S6 for schematic)—f-Ti 3 C 2 sheets. After a weak sonication of DMSO-intercalated f-MXene dispersed in deionized water, fully delaminated—that we denote as d-Ti 3 C 2 —flakes were obtained. After removal of large particles by centrifuging, the resulting aqueous colloidal solutions of d-MXene flakes were quite stable. The majority of flakes were small with a relatively narrow size distribution ( Fig. 4a ). The colloidal state of d-MXene flakes in aqueous solutions was also confirmed by the observation of the Tyndall scattering effect when passing a red laser beam through the solution (inset Fig. 4a ). SEM images clearly showed thin, electron-beam transparent, single MXene flakes precipitated from a drop of colloidal d-Ti 3 C 2 solution placed on a porous alumina membrane surface ( Fig. 4b ). 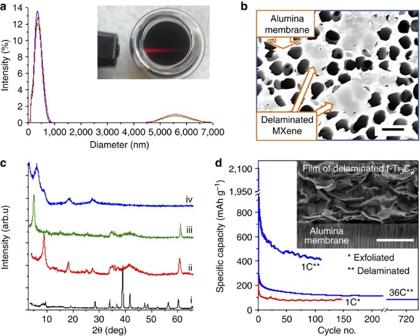Figure 4: Delaminated f-Ti3C2and its properties. (a) Particle size distribution in aqueous colloidal solution; inset shows Tyndall scattering effect in the solution. (b) SEM images of f-Ti3C2flakes on an alumina membrane. (c) XRD patterns of (i) Ti3AlC2, (ii) exfoliated, (iii) DMSO intercalated and (iv) delaminated Ti3C2. Note the disappearance of the non-basal peaks at ~60° in iv. (d) Comparison of the performance of exfoliated and delaminated f-Ti3C2as anode material in Li-ion batteries. Inset shows SEM image of an additive-free film of delaminated f-Ti3C2filtered through the membrane. Scale bars, 0.4 μm inb; 4 μm in insetd. Figure 4: Delaminated f-Ti 3 C 2 and its properties. ( a ) Particle size distribution in aqueous colloidal solution; inset shows Tyndall scattering effect in the solution. ( b ) SEM images of f-Ti 3 C 2 flakes on an alumina membrane. ( c ) XRD patterns of (i) Ti 3 AlC 2 , (ii) exfoliated, (iii) DMSO intercalated and (iv) delaminated Ti 3 C 2 . Note the disappearance of the non-basal peaks at ~60° in iv. ( d ) Comparison of the performance of exfoliated and delaminated f-Ti 3 C 2 as anode material in Li-ion batteries. Inset shows SEM image of an additive-free film of delaminated f-Ti 3 C 2 filtered through the membrane. Scale bars, 0.4 μm in b ; 4 μm in inset d . Full size image Binder-free MXene ‘paper’ (inset Fig. 4d ) was produced by filtering the aforementioned colloidal solution through a membrane. XRD patterns of the resulting ‘paper’ ( Fig. 4c ) clearly showed that the non-basal peaks at~60° 2θ vanished after delamination. This result provides compelling evidence for the loss of order along all, but [000l] and consequently, full delamination. Energy storage applications of delaminated MXene A recent computational study [25] concluded that d-Ti 3 C 2 layers would be attractive for Li-ion battery anodes. To date, our Li-ion work was carried out on stacked multilayer particles [23] , [24] . The breakthrough presented herein, however, allowed us to measure Li-ion uptake on d-Ti 3 C 2 ‘paper’. As shown in Fig. 4d , the capacity of the latter is a factor of 4 higher than that of as-synthesized f-MXene. The ‘paper’ showed a capacity of 410 mA h g −1 at a 1C cycling rate and 110 mA h g −1 at 36C ( Fig. 4d ). As shown in Supplementary Fig. S7 , the 410 mA h g −1 represents three Li per Ti 3 C 2 (OH) 2 . The capacity obtained at 1C was higher than the maximum theoretical capacity of f-Ti 3 C 2 MXene predicted by Tang et al . [25] using DFT (320 mA h g −1 ), although the as-delaminated d-MXenes have OH and F on the surface that theoratically reduce the reversible capacity. The reason for this mismatch is unclear at this time. However, a similar phenomenon observed on other nano-structured electrodes was explained by assuming the excess capacity stored in a unique reversible solid electrolyte interphase [31] , [32] , [33] , [34] , [35] . More work is ongoing to understand the lithiation and delithiation mechanisms of d-MXenes, in addition to further optimization of their performance. The results shown in Fig. 4d are noteworthy as they demonstrate Li capacities at 1C that are better than graphite, used in commercial LIBs. For example, at 280 mA h g −1 , graphite’s capacity at 1C is ≈75% of its theoretical capacity [36] . Similarly, lithium titanate is known for its capability to handle high cycling rates. For example, at 1C, the capacity of Li 4 Ti 5 O 12 was <170 mA h g −1 (ref. 37 ). Based on the results presented above, it is obvious that in ways reminiscent of graphite and clays, f-MXenes can be intercalated by a variety of organic molecules. This discovery can lead to the intercalation of a broad range of organics and salts, as well as provide routes to carry out complex chemical reactions—such as catalysis and polymerization (similar to intercalated graphite) [38] —within the f-MXene interlayer galleries. Furthermore, the intercalation of DMSO between f-Ti 3 C 2 sheets, followed by sonication in water, resulted in their delamination into separate sheets in an aqueous suspension from which a Ti 3 C 2 -based ‘paper’ was made. The Li uptake of the latter was significantly higher than its non-delaminated counterpart. The results obtained herein are of both fundamental and practical importance. On the fundamental side, they establish f-MXenes as full-fledged members of the growing family of 2D materials, with all the potential that such materials provide. It is crucial to note that in sharp contrast to most 2D materials made to date—in which weakly bonded layers were exfoliated/delaminated—the work presented here was carried out on the MAX phases, that are layered, but in which the bonding is exceptionally strong. Said otherwise, the world of 2D solids need not be restricted to layered solids with weak bonds, which is truly paradigm shifting. From a practical point of view, our results open avenues for the development of numerous applications in composites, catalysis, sorption and energy storage systems. Intercalation of f-MXene To intercalate f-MXene with HM, the f-MXene powders were suspended either in HM or a 1:3 mixture of HM and DMF, and magnetically stirred for 24 h , either at room temperature (RT) or at 80 °C. In all cases, the weight ratio of HM:MXene was 10:1. When the treatment involved only HM, the suspensions were filtered and washed with ethanol. In case of intercalation with HM/DMF mixture, DMF was used for washing instead of ethanol. The powders were then dried in a desiccator under vacuum (<10 Torr) at RT for 24 h or in the vacuum oven (~10 −2 Torr) at 120 °C for 24 h. Intercalation of other organic compounds was attempted. Those included DMSO, urea, DMF, acetone, ethyl alcohol, tetrahydrofuran, chloroform, toluene, thiophene and formaldehyde. In all cases, the intercalation procedure was the same: (i) 0.3 g of f-Ti 3 C 2 were mixed with 5 ml of each of the organic compounds listed above (excluding urea), then magnetically stirred for 24 h at RT; (ii) in the case of urea, 5 ml of 50 wt.% aqueous solution of urea was added to 0.3 g of f-Ti 3 C 2 and stirred for 24 h at 60 °C. Later, the resulting colloidal solutions were filtered and dried in a desiccator under vacuum (<10 Torr) at RT. A detailed experimental section (materials used, techniques of material preparation and de-intercalation of MXenes) can be found in the Supplementary Methods . De-intercalation of MXene To de-intercalate hydrazine/DMF, the intercalated MXene powder was carefully weighed, placed in a graphite crucible and outgassed at RT in vacuum (~10 −6 Torr) for 24 h. While under vacuum, the powder was then heated to 200 °C at 10 °C min −1 , held at this temperature for 72 h and cooled to RT. The powder remained under vacuum for another 48 h before it was retrieved. Between its removal from the furnace and re-weighing, the sample was exposed to ambient air for~3 min. Delamination of MXene For delamination, DMSO was used. After stirring of f-Ti 3 C 2 with DMSO for 18 h at room temperature, the colloidal suspension was centrifuged to separate the intercalated powder from the liquid DMSO. After decantation of the supernatant, deionized water was added to the residue in a weight ratio of f-MXene to water of 1:500. After bath sonication of the suspension for 6 h, centrifuging was carried out and the supernatant was filtered using a porous anodic aluminium oxide membrane filter (47 mm diameter, 0.2 μm pore size, Whatman Anodisc, Maidstone, UK) and dried in the oven at ~70 °C overnight, resulting in d-MXene ‘paper’ that detach easily from the membrane. Preparation of pressed MXene discs The non-intercalated and intercalated MXene powders were cold pressed under a load corresponding to a stress of 0.8 GPa using a manual hydraulic pellet press (Carver, Model 4350.L, Carver Inc., Wabash, USA). The resulting discs were 12.5 mm in diameter and 228–432 μm thick. Physical characterization XRD patterns were recorded with a powder diffractometer (Siemens D500, Germany) using Cu K α radiation (λ~1.54 Å) with 0.02° 2θ steps and 1 s dwelling time. A SEM (Zeiss Supra 50VP, Germany) was used to obtain images of the particles. The 2D sheets were also imaged with a TEM (JEOL JEM-2100, Japan) using an accelerating voltage of 200 kV. The TEM samples were prepared by suspending the powders in isopropanol, sonicating for 1 min and drying a drop of the mixture transferred on a 200 mesh lacey-carbon-coated copper grid. An XPS (PHI 5000, ULVAC-PHI Inc., Japan) was used to analyse the surface elemental composition of the powders before and after intercalation. The electrical resistance of cold-pressed discs of non-intercalated and intercalated MXenes was measured using a four-probe technique (Cascade Probe Station CPS-1303-24 with 4-point probe head Alessi C4S-57, Cascade Microtech Inc., Beaverton, USA). More information on techniques used for material characterization can be found in the Supplementary Methods . Electrochemical characterization Electrochemical measurements were carried out using coin cells. The lithium-ion batteries’ cyclabilities were studied using a galvanostatic charge-discharge cycling (GV) and a battery cycler (Arbin BT-2143-11U, College Station, TX, USA). In GV tests, the batteries were charged and discharged between 0 and 2.5 V versus Li/Li + with an imposed current, while the potential change was measured. From this measurement, the specific capacities were calculated for each cycle as Q =( I × t )/ m ; where Q is the specific capacitance (in mA h g −1 ), I is the current (in mA), t is the time (in h) and m is the mass of active material (in g). Note that for the f-MXene-based electrode before delamination, only the f-MXene mass, without that of the additives, was taken into account. For the delaminated d-MXene, as there were no additives, the mass considered is that of the d-MXene paper. Preparation of lithium coin cells The exfoliated, but un-delaminated, f-Ti 3 C 2 was made into an anode by mixing it with 10 wt.% poly(1,1-difluoroethylene) dissolved in 1-methyl-2-pyrrolidinone. The mixture was spread on Cu foil using a doctor blade, and dried at 140 °C for 12 h under vacuum (<10 Torr). To make the d-Ti 3 C 2 anode, dried ‘paper’ (3 mg cm −2 ) without any additives was used. Stainless steel coin cells, type CR-2016 (MTI, Richmond, CA, USA) were assembled with the f- or d-MXene as the positive electrode and Li metal foil as a counter electrode. A borosilicate glass fibre (Whatman GF/A, Buckinghamshire, UK) separated them. The electrolyte was a 1 M LiPF 6 solution in a 1:1 by weight mixture of ethylene carbonate and diethyl carbonate. The coin cells were assembled using crimping machine (MTI EQ-MSK-110, Richmond, CA, USA) in an Ar-filled glove box, with less than 1 p.p.m. of O 2 or H 2 O. MD simulations MD simulations were performed using Forcite module in Materials Studio suite (Accelrys). Owing to the unusual composition of the system, including C, Ti, O, N and H, the Universal Force Field [39] was used to calculate the system’s energy (see Supplementary Methods for details). Before simulations, 4 × 2 × 1 ( a × b × c ) OH-terminated Ti 3 C 2 periodic supercells with different numbers of N 2 H 4 molecules were constructed using the unit cell structure of f-Ti 3 C 2 from previous DFT simulations [17] . The supercells, subjected to isostatic external pressure of 0.1 MPa (1 atm), were first relaxed by geometry optimization (convergence tolerance: energy=0.02 cal mol −1 , force=1 cal mol −1 Å −1 , stress=1 MPa and displacement=0.00001 Å) with no constraints allowing for all atom positions in the cell, as well as the cell parameters, to be optimized. Charge distribution was calculated using the QEq method (initial charge=0, maximum iterations=100, convergence limit=0.0005 ē and parameter set=QEq_charged1.1). Once optimized, the supercells were used as initial structures in the MD runs. Constant number of particles N, pressure P, and temperature T (NPT) ensemble MD was performed at 298 K (Nose thermostat with Q ratio=1.0) with random initial velocities and 0.1 MPa external isostatic pressure (Berendsen barostat with decay constant=0.1 ps) for 300 ps with 1 fs steps (300,000 steps in total). Snapshots of the system were saved every 3,000 MD steps (100 snapshots in total) of which only the last 50 snapshots were used for analysis. This procedure allowed for >100 ps in the beginning of each run for thermal equilibration of the system with the analysis being performed on the part of MD trajectory corresponding to a system in an equilibrium state ( Supplementary Fig. S4b,c ), where all energy terms and density of the system remain nearly constant. No constrains on atom positions or cell parameters were applied during the MD run. During both the geometry optimization step and the MD run, the electrostatic interactions were summed up using Ewald scheme and the van der Waals interactions were summed up using the atom-based scheme. How to cite this article: Mashtalir, O. et al . Intercalation and delamination of layered carbides and carbonitrides. Nat. Commun. 4:1716 doi: 10.1038/ncomms2664 (2013).